Overcoming the brittleness of glass through bio-inspiration and micro-architecture Highly mineralized natural materials such as teeth or mollusk shells boast unusual combinations of stiffness, strength and toughness currently unmatched by engineering materials. While high mineral contents provide stiffness and hardness, these materials also contain weaker interfaces with intricate architectures, which can channel propagating cracks into toughening configurations. Here we report the implementation of these features into glass, using a laser engraving technique. Three-dimensional arrays of laser-generated microcracks can deflect and guide larger incoming cracks, following the concept of ‘stamp holes’. Jigsaw-like interfaces, infiltrated with polyurethane, furthermore channel cracks into interlocking configurations and pullout mechanisms, significantly enhancing energy dissipation and toughness. Compared with standard glass, which has no microstructure and is brittle, our bio-inspired glass displays built-in mechanisms that make it more deformable and 200 times tougher. This bio-inspired approach, based on carefully architectured interfaces, provides a new pathway to toughening glasses, ceramics or other hard and brittle materials. Many structural materials found in nature incorporate a large fraction of minerals to generate the stiffness and hardness required for their function (structural support, protection and mastication). In some extreme cases, minerals form more than 95% vol. of the material, as in tooth enamel [1] or mollusk shells [2] . With such high concentrations of minerals, one would expect these materials to be fragile, yet these materials are tough, durable, damage tolerant and can even produce ‘quasi-ductile’ behaviours. For example, nacre from mollusk shells is 3,000 times tougher than the mineral it is made of (in energy terms) [3] and it can undergo up to 1% tensile strain before failure, an exceptional amount of deformation compared to monolithic ceramics [4] . The question of how teeth, nacre, conch shell, glass sponge spicules, arthropod cuticles and other highly mineralized biological materials generate such outstanding performance despite the weakness of their constituents has been preoccupying researchers for several decades [3] , [4] , [5] , [6] , [7] . Bio-inspired concepts can open new pathways to enhancing the toughness of engineering ceramics and glasses, two groups of materials with very attractive properties, but whose range of applications is still limited by their brittleness [8] . In the recent years, an increasing number of synthetic composite materials inspired from biological materials have emerged, based on a wide range of fabrication techniques: ice templating [9] , [10] , layer-by-layer deposition/assembly [11] , [12] , [13] , self-assembly [14] , rapid prototyping [15] and manual assembly [16] . These new materials demonstrate that bio-inspired strategies can be harnessed to achieve both strength and toughness, two properties, which are typically exclusive [17] (for example, the strength of steel can be increased by cold working or increased carbon content, but this strengthening invariably comes with a decrease in ductility and toughness. Likewise, engineering ceramics are stiffer and stronger than metals, but their range of applicability is limited because of their brittleness). Despite the impressive properties displayed by some of these new bio-inspired materials, the level of ‘toughness’ amplification observed in natural materials is yet to be duplicated in synthetic composites. A transverse examination of how mineralized biological materials are constructed and how they fail reveals ‘universal’ rules, illustrated here with the examples of tooth enamel and nacre. The structure of these materials is organized over several distinct hierarchical length scales, from the nanoscale to the macroscale. Tooth enamel ( Fig. 1a ) is made of long rods perpendicular to the surface of the tooth and 4–8 μm in diameter [1] and held together by a small fraction of proteins (1% vol.). Similarly, nacre ( Fig. 1b ) is made of microscopic tablets of calcium carbonate [18] , with proteins and polysaccharides holding the structure together [19] . While these materials display features over several length scales, it appears that cracks preferentially interact with microscopic features. For example, cracks in nacre ( Fig. 1b ) propagate along the interfaces, circumventing the microscopic tablets and generating tortuous path, which dissipate more energy. The ability to guide and deflect cracks is fundamental to the performance of these materials, and it is only possible if the interfaces are weaker than the building blocks themselves [20] , [21] . The presence of weak interfaces may be perceived as detrimental to the performance of the material, but in fact it enables powerful toughening mechanisms. In tooth enamel, cracks typically emanate from the surface because of repeated contact or impact stresses. Initially, the cracks are channelled away from the surface and along the parallel rods, preventing chipping of the enamel surface. Deeper within enamel the rods bend and criss-cross, forming a complex decussation, which impedes further crack growth ( Fig. 1a ) [1] . More severe stresses may propagate the crack through the enamel layer where they meet another line of defence: the dentino-enamel junction [22] and underlying dentin [15] , [23] , [24] , [25] . Similarly, a crack propagating in nacre will be systematically deflected by the microscopic mineral tablets ( Fig. 1b ). Behind the crack tip, the tablets are still in contact and interact through the highly deformable interfaces [26] and associated nanoscale features [27] , [28] , exerting closure forces, which hinder crack propagation [29] . Furthermore, the wavy shape of the tablets generates progressive interlocking and progressive hardening at the local scale, so that tablet sliding propagates over large volumes around defects and cracks. These ‘process zones’ dissipate a tremendous amount of mechanical energy, which produces additional toughness [6] , [29] , [30] . 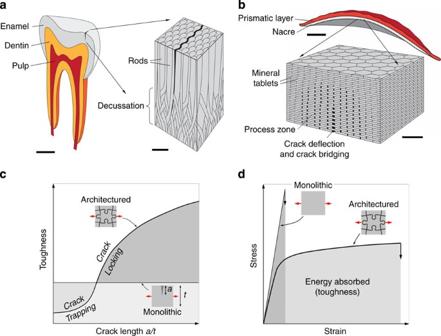Figure 1: Crack propagation and toughening mechanisms in natural materials. Crack propagation, crack channelling and toughening mechanisms in (a) tooth enamel (left scale bar: 2 mm, right scale bar: 10 μm) and (b) nacre (left scale bar: 20 mm, right scale bar: 5 μm). General concepts of weaker interface and architecture to generate (c) toughness and (d) large deformations and energy absorption.adenotes the length of a propagating crack andtdenotes width of the sample. Figure 1: Crack propagation and toughening mechanisms in natural materials. Crack propagation, crack channelling and toughening mechanisms in ( a ) tooth enamel (left scale bar: 2 mm, right scale bar: 10 μm) and ( b ) nacre (left scale bar: 20 mm, right scale bar: 5 μm). General concepts of weaker interface and architecture to generate ( c ) toughness and ( d ) large deformations and energy absorption. a denotes the length of a propagating crack and t denotes width of the sample. Full size image Mechanisms similar to those found in teeth and nacre have also been observed in cortical bone [31] , glass sponge spicules [32] and conch shells [33] , where crack deflection along microscopic features (osteons, lamellae and cross plies) dominates toughening mechanisms. The general concept found in these materials is illustrated in Figure 1c . Monolithic brittle materials display a low toughness of constant value, which does not change with crack advance a / t . The introduction of well-designed interfaces within the same material will completely change its mechanical response. Initially, crack propagation is induced along weak interfaces and around the building blocks, requiring little energy. On propagation a / t increases ( Fig. 1c ), and cracks are eventually channelled into configurations where additional mechanisms impede further propagation, effectively raising toughness, and trapping cracks into stable configurations. The ability of stabilizing cracks is essential for damage and flaw tolerance, reliability and durability. This type of material can also be described as building blocks with well-defined shapes and bonded by weaker interfaces, with similarities with emerging synthetic ‘architectured materials’ [34] . If the interfaces can sustain large deformations and dissipate energy, quasi-ductile behaviours may even be achieved in tension as observed in nacre and bone ( Fig. 1d ). In the deformation process, the interfaces play a central role, as they must absorb energy over large deformations [26] , [35] . In summary, nature uses three ‘overarching features’ to turn brittleness into toughness: (i) stiff and hard building blocks delimited by (ii) weaker interfaces arranged in (iii) specific architectures. In the present study we successfully implement these key features to turn glass, the archetype of a brittle material, into a tough and deformable material. Our approach consists of generating weak interfaces within the bulk of glass using three-dimensional laser engraving and infiltrating the interfaces with polyurethane. The weak interfaces channel the crack towards toughening configurations, which impede its propagation. The technique results in a bio-inspired glass that is 200 times tougher than the ‘intact’, non-engraved glass (throughout this article, by intact we refer to bulk glass, which was not engraved, but that is not devoid of the surface defects typical to glass exposed to air). Engraving weak interfaces within the glass bulk Lasers have been widely used in the past to alter the structure of materials and to generate useful structures at small scale and with high accuracy: surface roughness, microfluidic devices or waveguides [36] , [37] , [38] , [39] , [40] . Here we used a 3D laser engraving technique, which consists of focusing a laser beam at predefined points by using a set of two mirrors and a focusing lens ( Fig. 2a ). The UV laser beam (355 nm) used here travels in glass with little absorbance, and can be focused anywhere within the bulk of the material. When the system is properly tuned, the energy of the unfocused laser beam does not induce any structural changes in glass. However, the heat absorbed at the focal point is sufficient to generate radial microcracks from the hoop stresses associated with thermal expansion ( Fig. 2b ) [41] , [42] , [43] . These cracks only propagate over short distances, because the hoop stresses decrease rapidly away from the focal point. With a pulsed laser system, 3D complex arrays of thousands of defects can be engraved in a short period of time and with sub-micrometre precision ( Fig. 2c ). The size of the defects can also be tuned by adjusting the power of the laser. For our combination of glass material and laser (see Methods section) we found that a minimum average power of 35 mW is required to generate defects ( Fig. 2d ). Increasing the laser power generated larger cracks following a linear relationship, up to a plateau starting at a power of 140 mW. Powers beyond this threshold generated defects of constant size (about 25 microns). This response provided a window sufficiently large to tune the size of the microcracks. Arrays of such defects were then generated within the bulk of glass, effectively creating weaker interfaces following the concept of ‘stamp holes’: Once the weaker interfaces are engraved, the application of an external load may grow the microcracks until they coalesce, effectively channelling the propagation of long cracks. Furthermore, the toughness of the interface can be tuned by adjusting the size or spacing of the defects. To demonstrate these concepts we prepared compact tension fracture samples containing a pre-notch and an array of equi-spaced defects along the anticipated path of crack propagation ( Fig. 2e ). We used this geometry to measure the apparent toughness of the interface as function of defect size and spacing. 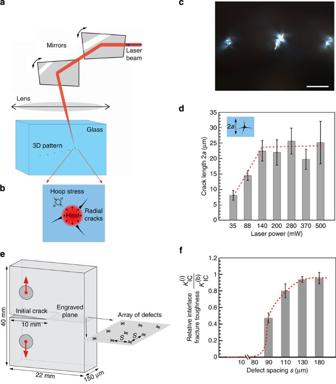Figure 2: Interfaces with tunable toughness by 3D laser engraving. (a) 3D laser engraving set-up. A laser beam is aimed and focused with high accuracy in the bulk of a block of glass. (b) The absorption of the energy provided by the laser raises the temperature locally, which generates hoop stresses and microcracks around the focal point. (c) Optical image of a line of micro-defects engraved within glass (scale bar: 50 μm).adenotes half the crack length. (d) The size of the micro-defects can be controlled by adjusting the power of the laser (the error bar corresponds to standard deviation,N=10 for each laser power). (e) Glass compact tension fracture specimen used to measure the fracture toughness of the engraved interface consisting of an array of micro-defects (spacings). (f) Effect of defect spacing on the fracture toughness of the interface (normalized by the fracture toughness of intact glass).andare the critical stress intensity factors of the interface and the bulk of the material, respectively. The error bars correspond to standard deviation (N=5 for each defect spacing). Figure 2f shows the effect of defect spacing on the toughness of the interface, for an average defect size of 25 μm. When these defects were very close to each other (spaced by 80 μm or closer), they coalesced on engraving without applying any external load, effectively cutting the sample in half (apparent toughness was zero). Increasing the spacing between the defects increased the toughness of the interface, up to a spacing of 130 μm. Defects more than 130 μm apart did not interact on application of an external load, and in these cases the apparent toughness was close to the toughness of intact glass (that is, no interface was created). These simple experiments show that 3D laser engraving can provide a fast and simple approach in generating weak interfaces of tunable toughness within glass. Figure 2: Interfaces with tunable toughness by 3D laser engraving. ( a ) 3D laser engraving set-up. A laser beam is aimed and focused with high accuracy in the bulk of a block of glass. ( b ) The absorption of the energy provided by the laser raises the temperature locally, which generates hoop stresses and microcracks around the focal point. ( c ) Optical image of a line of micro-defects engraved within glass (scale bar: 50 μm). a denotes half the crack length. ( d ) The size of the micro-defects can be controlled by adjusting the power of the laser (the error bar corresponds to standard deviation, N =10 for each laser power). ( e ) Glass compact tension fracture specimen used to measure the fracture toughness of the engraved interface consisting of an array of micro-defects (spacing s ). ( f ) Effect of defect spacing on the fracture toughness of the interface (normalized by the fracture toughness of intact glass). and are the critical stress intensity factors of the interface and the bulk of the material, respectively. The error bars correspond to standard deviation ( N =5 for each defect spacing). Full size image Guiding cracks along engraved interfaces Our next step was to exploit these weak interfaces in order to deflect and channel cracks along predefined paths. Theoretical fracture mechanics predicts that an incident crack propagating in mode I (opening) intersecting a weak interface at an angle θ may either deflect along the interface or proceed into the bulk of the material ( Fig. 3a ). 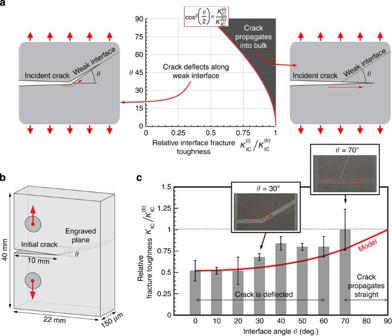Figure 3: Crack deflection into weak interfaces. (a) An incident crack intersects a weaker interface at an angleθ. On applying tensile stress, theoretical fracture mechanics predicts that the crack may be deflected along the weaker interface or ignore the weaker interface and propagate straight into the bulk of the material.andare the critical stress intensity factors of the interface and the bulk of the material, respectively. (b) Glass compact tension fracture sample used to assess channelling of cracks in glass. (c) The apparent toughness increases as the crack is deflected. Past a critical angle, in this case 70°, the crack ignores the weak interface and propagates straight. The fracture toughness is then that of intact glass (the fracture toughness of interface is half the toughness of intact glass). The experiments agree well with the theoretical predictions. The error bars give the standard deviation of the relative fracture toughness (N=5 for each angle). The condition for the crack to propagate and deflect into the weak interface may be written in energy terms [44] : Figure 3: Crack deflection into weak interfaces. ( a ) An incident crack intersects a weaker interface at an angle θ . On applying tensile stress, theoretical fracture mechanics predicts that the crack may be deflected along the weaker interface or ignore the weaker interface and propagate straight into the bulk of the material. and are the critical stress intensity factors of the interface and the bulk of the material, respectively. ( b ) Glass compact tension fracture sample used to assess channelling of cracks in glass. ( c ) The apparent toughness increases as the crack is deflected. Past a critical angle, in this case 70°, the crack ignores the weak interface and propagates straight. The fracture toughness is then that of intact glass (the fracture toughness of interface is half the toughness of intact glass). The experiments agree well with the theoretical predictions. The error bars give the standard deviation of the relative fracture toughness ( N =5 for each angle). Full size image Where, G (i) and G (b) denote the energy release rate of the weak interface and the bulk material, respectively, and G c (i) and G c (b) are the critical energy release rates for the interface and the bulk of the material. G c (i) and G c (b) are material properties, which are measured experimentally. Here they are given by: Where, E ′= E for plane stress and E ′= for plane strain. E and v denote Young’s modulus and Poisson’s ratio of the material. and are the critical stress intensity factors (fracture toughness) of the interface and the bulk of the material. The incident crack is in mode I and its stress intensity factor is denoted by K I . We only consider pure mode I for the incident crack so that K II =0. The associated bulk strain release rate is then: Meanwhile, since the interface is slanted it undergoes mixed mode loading, with stress intensity factors [45] : The associated strain energy release rate is then: Combining equations 1, 2, 3 and 5, the condition for the crack to propagate into the interface becomes: This criterion is illustrated in Figure 3a : crack deflection can be achieved if the toughness of the interface is sufficiently low relative to the toughness of the bulk material, and provided that the deflection angle θ is not too large. If the crack indeed propagates along the interface, then the crack enters a mixed mode condition, which will lead to an increase in apparent toughness K c following: Here we implemented these principles by deflecting cracks into weak interfaces engraved in glass. Our fracture specimens consisted of an initial crack and an engraved plane of equi-spaced defects ahead of the crack tip, tailored to have half of the toughness of bulk glass. The interface was positioned at different angles θ from the initial crack plane ( Fig. 3b ). In the experiments the interface could deflect the crack up to an angle of θ =60° ( Fig. 3c ). At θ =70° and above the crack propagated straight into the bulk of the material. As predicted by the model, the apparent toughness increased with higher angle, from half of the toughness of glass at θ =0° up to the toughness of glass at θ =70° ( Fig. 3c ). Channelling cracks into toughening configurations The ability to guide cracks within glass can be exploited to channel cracks into configuration where propagation becomes more difficult, which is the strategy observed in enamel and nacre. Here, we engraved a weak interface with jigsaw-like features ahead of an incident crack. This intricate line, reminiscent of sutures in some natural materials [46] , consisted of a periodic repetition of tabs with round features to limit stress concentrations ( Fig. 4a ). Arcs of circle (radius R ) interpenetrated and formed re-entrant locking features with locking angle θ 0 ( Fig. 4b ). By tuning the laser power (110 mW) and the spacing of the defects (Methods section), we ensured that the crack propagated through the engraved interfaces. This initial propagation, relatively easy, revealed a second line of mechanism: as the tabs were pulled apart they progressively interlocked, as an increasing amount of traction was necessary to overcome the normal contact forces and friction ( Fig. 4c ). We implemented this jigsaw-like interface ahead of a crack in a glass sample ( Fig. 4d ) with R =0.5 mm and θ 0 =5°. Crack propagation was very stable, and was dominated by the pullout of the jigsaw tabs ( Fig. 4e ). The corresponding force-opening curve ( Fig. 4f ) had a bell-shape characteristic of stable crack propagation in tough materials. We then used an integration method to obtain the traction-separation curve of the interface from the force-opening curve [47] (Methods section). 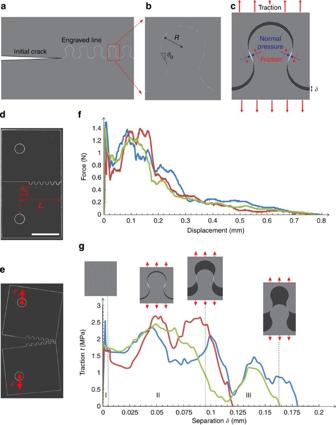Figure 4: Stable crack propagation into toughening configurations. (a) A jigsaw-like interface is engraved in front of the main crack. (b) The basic geometrical motif can be characterized by the radiusRand the locking angleθ0. (c) When the crack propagates along the engraved interface the jigsaw tab is pulled out by a distanceδ, and normal pressures and frictional tractions develop. (d) Actual glass fracture sample at rest (scale bar: 10 mm) and (e) after the test.Fis the pulling force,Lis the distance from the line of action of the pulling force to the end of the engraved line, anda0is the initial crack length. (f) Force-displacement curves for the jigsaw interface showed stable crack propagation. (g) The experiment yield the traction-separation curve, or cohesive law, for the interface obtained from the original force-displacement curve using an integration method. Figure 4g shows typical traction-separation curves: the initial response (stage I) is linear elastic up to about 2 MPa, at which point the interface fails in a brittle fashion (sudden drop). The traction increases again but at a lower slope (stage II), corresponding to the progressive pullout and interlocking of the jigsaw features. When the traction reaches its maximum (2.5 MPa), the contact pressures are perpendicular to the pullout direction and therefore do not contribute to pullout resistance. There is still, however, a large resistance to pull generated by friction, so that the locking tabs still provide a decreasing but non-negligible traction in stage III ( Fig. 4g ). The traction finally vanishes when the two tabs are completely pulled apart, at a separation distance of about 0.15 mm. Figure 4: Stable crack propagation into toughening configurations. ( a ) A jigsaw-like interface is engraved in front of the main crack. ( b ) The basic geometrical motif can be characterized by the radius R and the locking angle θ 0 . ( c ) When the crack propagates along the engraved interface the jigsaw tab is pulled out by a distance δ , and normal pressures and frictional tractions develop. ( d ) Actual glass fracture sample at rest (scale bar: 10 mm) and ( e ) after the test. F is the pulling force, L is the distance from the line of action of the pulling force to the end of the engraved line, and a 0 is the initial crack length. ( f ) Force-displacement curves for the jigsaw interface showed stable crack propagation. ( g ) The experiment yield the traction-separation curve, or cohesive law, for the interface obtained from the original force-displacement curve using an integration method. Full size image We also computed the toughness of the interface, which is given by the area under the traction-separation curve (which, in this case, represents the energy dissipated by friction over the unit area of the crack). In this case, nonlinear dissipative mechanisms such as friction play an important role in generating toughness, and therefore the toughness measured corresponds to J IC , a commonly used measure of toughness in nonlinear fracture mechanics [48] (if the material is linear elastic then J IC is equal to the strain energy release rate [48] ). The area under the traction-separation curve yielded a toughness of 200±17 J m −2 for a locking angle of θ 0 =5°. For comparison, intact glass has a toughness of only about 3 J m −2 (ref. 49 ). The toughness of the engraved glass can be even further increased by increasing the locking angle ( Fig. 5c ): increasing θ 0 from 5 to 7° initially increased the toughness and strength of the interface, and the highest toughness we produced was 360±80 J m −2 at a locking angle of θ 0 =5.5°. This material is more than 100 times tougher than intact glass, an unprecedented amplification of toughness for this type of material. Beyond θ 0 =5.5° the toughness decreases because of excessive damage to the glass tabs ( Fig. 5a,b ). 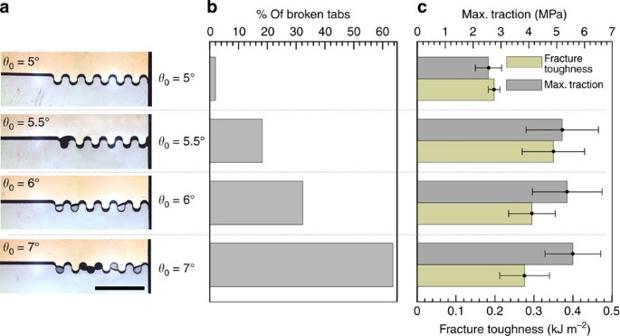Figure 5: Tuning the locking angle for toughness amplification in bio-inspired glass. The resulting design is a trade-off between maximizing toughness and minimizing damage to the tabs: (a) actual pictures of fractured samples with increasing locking angleθ0(scale bar: 6 mm); (b) fraction of tabs broken during the test; (c) maximum traction and toughness as function of locking angle (the error bars correspond to standard of the measured property,N=5 for each angle). Figure 5: Tuning the locking angle for toughness amplification in bio-inspired glass. The resulting design is a trade-off between maximizing toughness and minimizing damage to the tabs: ( a ) actual pictures of fractured samples with increasing locking angle θ 0 (scale bar: 6 mm); ( b ) fraction of tabs broken during the test; ( c ) maximum traction and toughness as function of locking angle (the error bars correspond to standard of the measured property, N =5 for each angle). Full size image Engraved glass infiltrated with polyurethane We further improved the performance of our bio-inspired material by infiltrating the interfaces with a low-viscosity polyurethane. We measured the cohesive law of the polyurethane on straight interface ( Fig. 6a ), corresponding to a fracture toughness of 200 J m −2 . We then measured the cohesive response of engraved glass samples infiltrated with polyurethane ( Fig. 6a ). The fracture toughness of the infiltrated samples was 600±110 J m −2 , which is 200 times the toughness of the intact glass, 1.6 times the toughness of the non-infiltrated engraved glass and three times the toughness of polyurethane on straight interface. Cross-linked polyurethane is an elastomer, which provided cohesive strength to the material over large opening distances, by the formation of ligaments reminiscent of the ligaments formed by organic materials at the interfaces of natural materials [50] ( Fig. 6b ). The adhesive finally served as a ‘soft cushion’ that reduced the severity of stresses at the contact region between the neighbouring tabs. We could therefore increase the optimum angle from 5.5° (for the not-infiltrated interfaces) to 7° for the interfaces infiltrated with polyurethane, which led to a tensile strength of about 10 MPa. Engraved glasses infiltrated with other types of adhesives were not successful: Polydimethylsiloxane (PDMS) was too weak and did not improve the performance of the material significantly. On the other hand, cyanoacrylate was too stiff and strong, and the crack did not follow the engraved pattern, leading to a catastrophic failure. 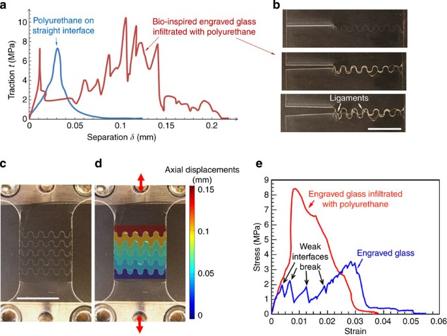Figure 6: Bio-inspired architecture infiltrated with polyurethane. (a) Traction-separation curves for polyurethane on straight interface and for the engraved glass infiltrated with polyurethane. (b) Progressive opening of the engraved glass interface infiltrated with polyurethane, showing ligaments (scale bar: 4 mm). (c) Image of an actual tensile sample at the start of the test and (d) at the maximum tensile force, with displacements obtained with image correlation (scale bar: 8 mm). (e) Typical stress-strain curves of the engraved and engraved-infiltrated glass with five parallel jigsaw-like sutures. The arrows indicate the drops in stress corresponding to the sequential fracture of the engraved interfaces. Figure 6: Bio-inspired architecture infiltrated with polyurethane. ( a ) Traction-separation curves for polyurethane on straight interface and for the engraved glass infiltrated with polyurethane. ( b ) Progressive opening of the engraved glass interface infiltrated with polyurethane, showing ligaments (scale bar: 4 mm). ( c ) Image of an actual tensile sample at the start of the test and ( d ) at the maximum tensile force, with displacements obtained with image correlation (scale bar: 8 mm). ( e ) Typical stress-strain curves of the engraved and engraved-infiltrated glass with five parallel jigsaw-like sutures. The arrows indicate the drops in stress corresponding to the sequential fracture of the engraved interfaces. Full size image Performance in uniaxial tension These interfaces and locking mechanisms can be repeated periodically within the bulk of glass delaying localization and dissipating energy over large volumes. Figure 6c shows a tensile glass sample with five jigsaw-like interfaces ( R =0.5 mm, θ 0 =7°, spacing=1.75 mm), and Figure 6e shows the corresponding tensile stress-strain curves. For the case of non-infiltrated interfaces the sudden drops in stress correspond to an interface failing, followed by a raise in the stress due to the progressive locking mechanism. The locking was strong enough to raise the stress to a level sufficient to fail other interfaces in the material, thus propagating the pullout process over large volumes (which is a key mechanism in nacre [4] , [6] ). Eventually every jigsaw feature was pulled out ( Fig. 6d ), and the stress kept increasing with deformation with small fluctuations in load associated with dry friction. This failure mode duplicated some of the most remarkable features of natural nacre: delocalization of deformations over large volumes, ductile-like deformation and damage tolerance. When the stress reached the maximum traction at one of the interfaces, the material became unstable, deformation eventually localized and the stress decreased with deformation. These weaker interfaces, properly designed and tuned, therefore turned brittle glass into a deformable material failing at almost 5% strain. Infiltrating the engraved glass with polyurethane had two effects on the tensile response. The failure and pullout were smoother because of the ‘cushion effect’ and the formation of ligaments discussed above, and the material was also significantly stronger, reaching a tensile strength of about 8–9 MPa. The area under the stress-strain curve gives the energy dissipated by the material per unit volume, corresponding to 70 kJ m −3 and 130 kJ m −3 for the non-infiltrated and infiltrated materials, respectively. For comparison, four-point bending tests on the intact borosilicate glass slides used here revealed a modulus of 62.5 GPa and flexural strength of 80–100 MPa, which is 10 times higher than our engraved glass. The strain at failure of intact glass was 0.0017, about 20 times less than the strain at failure of the engraved material. Finally, the strain energy of intact glass just before failure was 50–80 kJ m −3 but because of the catastrophic fracture of glass, only a small portion of the stored strain energy is actually consumed by the formation of cracks (most of the energy being dispelled in dynamic effects and other propagations to connective components [51] ). The engraved glass has lower strength than intact glass, which was expected; an improvement in toughness and ductility is generally accompanied with a decrease in strength. In comparison, while the tensile strength of the mineral tablets in nacre has never been measured experimentally, it can be estimated using fracture mechanics, using [49] : With ≈0.39 Mpa m 1/2 as the toughness of the mineral [52] and a ≈30 nm as the size of the defects within the tablets one finds a tensile strength in the order of 1 GPa. For comparison, the tensile strength of nacre is about 10 times lower, in the order of 100 MPa. The strength of nacre is controlled by shearing of the soft interfaces between the tablets, and the apparent strength of the tablets is much lower than 1 GPa, because of stress concentrations arising from the staggered arrangement [53] . The decrease in strength in nacre compared with pure mineral is therefore in the same order as the decrease in strength in our material compared with intact glass. Highly mineralized natural materials owe their exceptional properties to microscopic building blocks, weak interfaces and architecture. Making a material tougher by introducing weak interfaces may seem counterintuitive, but it appears to be a universal and powerful strategy in natural materials. Here we demonstrate, using 3D laser engraving, that this approach is indeed exceptionally powerful. By fine-tuning the toughness and structure of the interfaces, we amplified the toughness of glass by a factor of 200, and turned it into a deformable material failing at almost 5% strain. The locking angle of the tabs is a critical parameter in the optimization of the material. Higher overall strength and toughness could be produced with larger angles, but the angle must be kept within limits to prevent the fracture of the locking tabs themselves. The fracture toughness of the bulk material and the size of the defects generated by the engraving process are therefore important factors to take into account if other types of glasses or ceramics were considered as base materials. One can also envision the exploration of more complex 3D structures inspired by nature. The laser engraving technique offers a powerful approach in generating intricate 3D microstructures with accuracy, which can be finely tuned to obtain desirable combinations of strength and toughness. While in this work we focused on millimeter-sized features to demonstrate key mechanisms, the fabrication method can also be scaled down to the micro and nanometre length scales using femtosecond lasers [36] . Reducing the size of the structure will enable higher overall strength, following scaling principles observed in nature [54] . Fabrication of the fracture test samples 150 μm-thick rectangular (22 × 40 mm) optical grade 263 M borosilicate glass slides (Fisher Scientific Catalogue NO. 12545C, Ottawa, ON) were engraved using a 3D laser engraver (Model Vitrolux, Vitro Laser Solutions UG, Minden, Germany) equipped with a pulsed UV laser (355 nm, 0.5 W cw pumped, 4 kHz repetition rate, 4–5 ns pulse duration). The slide was cut down to a 22 mm × 40 mm plate using the laser in ‘cutting mode’ with a power of 500 mW and defect spacing of 5 μm. Pin holes and initial notch were prepared using the same procedure. A weaker interface consisting of an array of defects was then engraved ahead of the initial notch. The toughness of the interface was tuned by adjusting the laser power and/or the spacing between the defects. For engraving the tilted weak interfaces ahead of the crack tip, power and defect spacing of 200 mW and 90 μm were used, respectively. This combination of power and defect spacing resulted in an interface with half the toughness of the bulk glass. For engraving the weak jigsaw-like interfaces, the power of the laser was reduced to 110 mW. In order to improve the stiffness and strength of the tabs, the engraved patterns were divided into two regions: at contact regions between the neighbouring tabs where the locking and the friction occur, higher defect spacing of 2.75 μm was used. This approach decreased the amount of damage to the tabs at contact regions, and increased the interface stiffness and strength. For the rest of the interface, lower defect spacing of 2.5 μm was used so that the crack would be able to follow the interface. The defects were equi-spaced in both in-plane and out-plane directions. The sample geometry for the jigsaw-like fracture specimens and fracture specimens with tilted weak interface were the same (150 μm-thick rectangle 22 mm × 40 mm). For infiltrated samples, polyurethane adhesive (U-09FL, Loctite, CT, USA) was used. All samples were tested using a miniature loading machine (Ernest F. Fullam Inc., Latham, NY, USA) at a displacement rate of 3 μm s −1 . All the tests were performed in the ‘Biomimetic lab’ at McGill University at which the humidity is controlled in the range of 30–35%. The tensile specimens were prepared using a similar method and by repeating the engraving jigsaw-like interfaces five times and across the entire width of the sample. Determination of traction-separation curves Following the Rigid Double Cantilever Beam method developed by Khayer Dastjerdi et al . [48] and by considering negligible elastic deformation within the intact glass material, the interface separation δ and the traction t , which are generated through interlocking of jigsaw-like features can be obtained using: Where, L is the distance from the line of action of the pulling force F to the end point of the engraved line, B is the thickness of the glass specimen, a 0 is the initial crack length, and Δ is the opening at the loading line ( Fig. 4d ). Equation 9 was used to obtain the traction-separation curves from the experimentally obtained force-displacement ( F −Δ) data for the jigsaw-like interfaces. How to cite this article: Mirkhalaf, M. et al . Overcoming the brittleness of glass through bio-inspiration and micro-architecture. Nat. Commun. 5:3166 doi: 10.1038/ncomms4166 (2014).